Huge critical current density and tailored superconducting anisotropy in SmFeAsO0.8F0.15by low-density columnar-defect incorporation Iron-based superconductors could be useful for electricity distribution and superconducting magnet applications because of their relatively high critical current densities and upper critical fields. SmFeAsO 0.8 F 0.15 is of particular interest as it has the highest transition temperature among these materials. Here we show that by introducing a low density of correlated nano-scale defects into this material by heavy-ion irradiation, we can increase its critical current density to up to 2 × 10 7 A cm −2 at 5 K—the highest ever reported for an iron-based superconductor—without reducing its critical temperature of 50 K. We also observe a notable reduction in the thermodynamic superconducting anisotropy, from 8 to 4 upon irradiation. We develop a model based on anisotropic electron scattering that predicts that the superconducting anisotropy can be tailored via correlated defects in semimetallic, fully gapped type II superconductors. The reasonably high values of the superconducting transition temperature T c , very high upper critical magnetic fields and generally low anisotropy of the recently discovered iron-based superconductors [1] , [2] , [3] enable operation in economically interesting temperature-field ranges and, at the same time, minimize detrimental effects due to grain boundaries and thermal fluctuations [4] , [5] . However, the overriding application metric, the maximum loss-less electrical current density, is ultimately determined by the vortex pinning that can be engineered into the material. Significant advances towards high-performing superconducting materials based on the so-called 122-compounds, most notably Ba(Fe 1− x Co x ) 2 As 2 and Ba 1− x K x Fe 2 As 2 (refs 6 , 7 , 8 ), and 11-compounds [9] have been made. For instance, Ba 0.6 K 0.4 Fe 2 As 2 has demonstrated a nearly field-independent critical current density of J c =5 MA cm −2 at 5 K and H~7 T (ref. 10 ). These J c (T,H) values are comparable to state-of-the-art YBa 2 Cu 3 O 7- δ (YBCO)-coated conductors under similar conditions. However, the relatively low values of T c , 23 and 38 K, respectively, pose serious limitations. FeAs-1111 compounds, such as SmFeAsO 1− x F x , have T c in excess of 50 K (ref. 11 ). In addition, high critical current densities approaching 1–2 MA cm −2 in as-grown SmFeAsO 1− x F x crystals and films at 5 K and self-field have been reported [12] , [13] , [14] . However, the layered structure of SmFeAsO 1− x F x , shown in Fig. 1a , leads to a rather high anisotropy, γ ~8 (refs 15 , 16 ), exceeding that of YBCO, which causes the suppression of the irreversibility field and limitation of applications at high fields and high temperature. To mitigate these drawbacks, nano-scale columnar defects in optimal-doped SmFeAsO 0.8 F 0.15 crystals were produced. Columnar defects have been proven very effective in vortex pinning in high- T c cuprates [17] as they are capable of trapping vortices over extended sections of their length (see Fig. 1b ). To date, the performance of SmFeAsO 0.8 F 0.15 with columnar pinning landscape is unknown, and the ceiling of J c of the iron-based superconductors remains an open question. 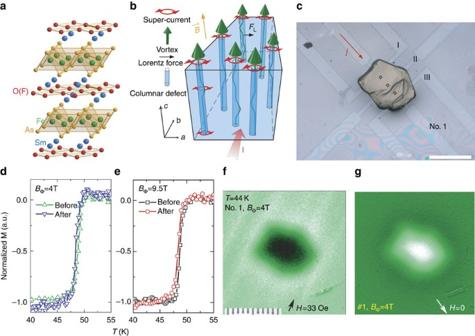Figure 1: Heavy-ion-irradiated SmFeAsO0.8F0.15and magnetization characterizations. aandbare schematic pictures of the layered structure of SmFeAsO1−xFxand of the correlated nano-scale defects produced by the high energy, heavy-ion irradiation. (c) Image of sample no. 1 placed on top of a micro-Hall array magnetometer. The black open squares represent the position of the individual Hall-probe sensing areas underneath the crystal. (d) and (e) Magnetization measurements of sample no. 1 and no. 2, pre- and post irradiation.Tcremains virtually unchanged following irradiation. (f) and (g) Magneto-optical imaging of magnetic flux in sample no. 1 in increasing and decreasing applied magnetic fields. The scale bars in (c) and (f) represent 100 μm. Figure 1: Heavy-ion-irradiated SmFeAsO 0.8 F 0.15 and magnetization characterizations. a and b are schematic pictures of the layered structure of SmFeAsO 1− x F x and of the correlated nano-scale defects produced by the high energy, heavy-ion irradiation. ( c ) Image of sample no. 1 placed on top of a micro-Hall array magnetometer. The black open squares represent the position of the individual Hall-probe sensing areas underneath the crystal. ( d ) and ( e ) Magnetization measurements of sample no. 1 and no. 2, pre- and post irradiation. T c remains virtually unchanged following irradiation. ( f ) and ( g ) Magneto-optical imaging of magnetic flux in sample no. 1 in increasing and decreasing applied magnetic fields. The scale bars in ( c ) and ( f ) represent 100 μm. Full size image Here we incorporated a low density of columnar defects into pristine SmFeAsO 0.8 F 0.15 crystals using high-energy, heavy-ion irradiation along the c-axis. The induced columnar defects produce record-high values of the critical current density without degradation of the transition temperature. The enhanced critical current to J c (5 K, 0 T)≈20 MA cm −2 corresponds to ~20% of the depairing current. Furthermore, we found a pronounced reduction in the superconducting anisotropy from 8 to 4 following the irradiation. Such a phenomenon can be qualitatively understood in the framework of anisotropic electron scattering by columnar defects. Columnar-defect incorporation SmFeAsO 0.8 F 0.15 single crystals with an approximate size of 100 × 100 × 6 μm 3 (shown in Fig. 1c ) and submicrogram mass were grown at ETH Zurich in a high-pressure synthesis procedure using NaCl/KCl flux [18] , [19] . Two SmFeAsO 0.8 F 0.15 crystals were irradiated at the ATLAS facility at Argonne National Laboratory with 1.4-GeV Pb –ions to doses of N =2 × 10 11 (sample no. 1) and 5 × 10 11 ions cm −2 (sample no. 2), corresponding to nominal dose-matching fields of B Φ =4 and 9.5 T along the crystal’s c-axis; B Φ = NΦ 0 , where Φ 0 =2.07 × 10 15 Tm 2 . Heavy-ion irradiation leaves amorphous tracks (columnar defects) where the ions have traversed through the sample [20] . Compared with the structural density of 6 × 10 14 unit cells cm −2 for SmFeAsO 0.8 F 0.15 , the concentration of tracks is rather dilute, ~2–5 tracks per 1,000 unit cells. Transition temperatures Figure 1d,e shows SQUID magnetic measurements in a field of 1 Oe ( H //c) after zero-field cooling for the two SmFeAsO 0.8 F 0.15 crystals before and after irradiation. We observe a temperature-independent magnetic moment at low temperatures and a sharp superconducting transition at T c =50 K with ΔT c ~1.5 K, underlining the high quality of the crystals. Our results show that the transition temperature and transition width do not change appreciably for irradiation doses up to 9.5 T. Similar robust transition temperatures against heavy-ion-induced defects were observed in Ba 0.6 K 0.4 Fe 2 As 2 crystals with 1.4-GeV Pb-ion irradiation doses up to B Φ =21 T (ref. 10 ). These results suggest that in both, the FeAs-1111 and the FeAs-122-compounds, columnar defects induce non-magnetic small-angle intra-band scattering, which does not contribute to pair-breaking for s ± -gap symmetry. Critical current densities The small size of the crystals used in our study precludes the use of a commercial SQUID magnetometer to obtain J c through magnetic hysteresis measurements at temperatures above 20 K. We therefore placed the crystal onto a highly sensitive micro-Hall-array magnetometer (see Fig. 1c ). The crystal was carefully aligned with a high precision manipulator to ensure that the same position within 5 μm was maintained for measurements before and after irradiation, corresponding to an uncertainty of <10%. The black squares in Fig. 1c denote the three active areas of the Hall-array, with the middle sensor located at the centre of the crystal. A magneto-optical (MO) indicator film technique [21] was used to check for weak links such as grain boundaries in the samples. The images of field screening and trapped flux after switching off the external magnetic field are shown in Fig. 1f,g for sample no. 1. No weak-link areas for preferential entry/exit of vortices can be detected, confirming the single grain and homogeneous critical current density behaviour over the entire sample. 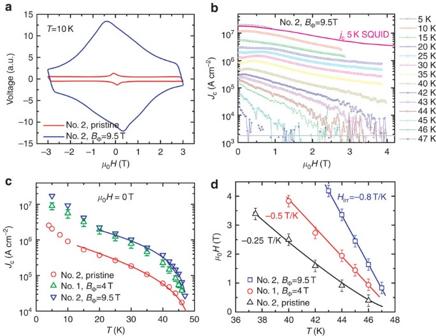Figure 2: Critical current density and irreversibility field of irradiated SmFeAsO0.8F0.15. (a) Micro-Hall-bar voltage signal from the middle sensor for sample no. 2 before and after irradiation to a dose-matching field ofBΦ=9.5 T. (b) Magnetic field dependence ofJcat various temperatures for sample no. 2. The magenta solid line is theJcdetermined from SQUID measurements atT=5 K using the Bean model calculation. The open symbols areJcobtained from the micro-Hall-array magnetometer. (c)Jcas a function of temperature for the pre-irradiated sample no. 1, postirradiated sample no. 1 (BΦ=4 T) and sample no. 2 (BΦ=9.5 T). 10%Jcuncertainty of postirradiated sample no. 1 arises from the different determinations between measurements of Hall array and magneto-optical imaging. (d) The irreversibility line for the investigated three samples.Jc=2,000 A cm−2was used as a criterion to determine the irreversibility fields. Uncertainty comes from the noise inJcmeasurement which is shown inb. The solid lines incanddare guides to the eye. Figure 2a compares the magnetic hysteresis loops at the centre of sample no. 2 at T =10 K before and after irradiation to a dose of B Φ =9.5 T. A ten-fold enhancement can be observed for the irradiated sample. This large enhancement factor is observed over the entire temperature range from T =5 to 40 K. For comparison between local and global magnetization measurements, we measured the magnetization hysteresis curve of sample no. 2 with a SQUID magnetometer at T =5 K, where the signal was large enough to be detected from the small crystals. Using the Bean model [22] J c =20 ΔM/a (1 -a /3 b ), we obtained J c values from the hysteresis loop width, ΔM . A calibration factor was obtained by comparing the J c value determined by SQUID magnetometry at low temperature and the J c values obtained from the micro-Hall-array magnetometer. This factor was used to convert the micro-Hall-array data to J c values at high temperatures. The derived J c (H,T) -values for the 9.5-T-irradiated sample no. 2 at various temperatures and fields are presented in Fig. 2b . At 5 K and self-field, the critical current density is remarkably high J c =1.8~2 × 10 7 A cm −2 , whereas J c at 44 K and 0 T is 2 × 10 5 A cm −2 . As for the 4 T-irradiated sample no. 1, the critical current derived using the same method yields J c =9 × 10 6 A cm −2 at 5 and 0 T, ~4.5 times the J c (5 K, 0 T) of the pristine sample. The depairing current of SmFeAsO 0.85 F 0.15 can be estimated by , where Φ 0 is the flux quantum, and using values of the penetration depth λ ~200 nm and the coherence length ξ ab (0)~1.5 nm (refs 2 , 16 , 23 ). The calculated value of j 0 ~1 × 10 8 A cm −2 indicates that we have achieved ~20% of the depairing current by simply incorporating a low density of columnar defects. To the best of our knowledge, such a high J c value has not been reported on any of the iron-based superconductors. This is a remarkably high J c for a single crystal, considering that even in state-of-the-art YBCO conductors, the self-field J c has reached only 15–25% of the depairing current after a decade of pinning landscape engineering [24] , [25] , [26] . By increasing the density of defects and by combining different types of pinning centres into SmFeAsO 0.8 F 0.15 , further enhancement of J c can be expected. Figure 2: Critical current density and irreversibility field of irradiated SmFeAsO 0.8 F 0.15 . ( a ) Micro-Hall-bar voltage signal from the middle sensor for sample no. 2 before and after irradiation to a dose-matching field of B Φ =9.5 T. ( b ) Magnetic field dependence of J c at various temperatures for sample no. 2. The magenta solid line is the J c determined from SQUID measurements at T =5 K using the Bean model calculation. The open symbols are J c obtained from the micro-Hall-array magnetometer. ( c ) J c as a function of temperature for the pre-irradiated sample no. 1, postirradiated sample no. 1 ( B Φ =4 T) and sample no. 2 ( B Φ =9.5 T). 10% J c uncertainty of postirradiated sample no. 1 arises from the different determinations between measurements of Hall array and magneto-optical imaging. ( d ) The irreversibility line for the investigated three samples. J c =2,000 A cm −2 was used as a criterion to determine the irreversibility fields. Uncertainty comes from the noise in J c measurement which is shown in b . The solid lines in c and d are guides to the eye. Full size image Figure 2c shows the temperature dependence of J c before and after irradiation. The order-of-magnitude enhancement of J c due to irradiation is apparent over the entire temperature range. The initial (almost) exponential decrease of J c with temperature followed by a power-law variation has been observed for several 1111-materials [27] . It has been suggested that at low field (self-field) and low temperatures, strong single-vortex pinning is dominant [27] , whereas at higher temperature, effects due to collective pinning and creep become important. Using a criterion of J c =2 × 10 3 A cm −2 , we determined the irreversibility line H irr . The slope of H irr increases by a factor of 2–3 after irradiation, as shown in Fig. 2d . These results demonstrate that a low density of columnar defects can firmly pin the vortices and effectively extend the useful range in the H – T phase diagram into the vortex liquid region. Thermodynamic superconducting anisotropy and model Another remarkable aspect of columnar defects is the surprising reduction of the thermodynamic superconducting anisotropy. Here, we use a highly sensitive membrane-based steady-state ac micro-calorimeter to measure the specific heat of the submicrogram crystals [28] and to determine the superconducting anisotropy. The specific heat anomaly near T c ~50 K of sample no. 1 in zero field is delineated in Fig. 3a . Subtraction of the normal state background as described in detail in Welp et al . [16] yields the superconducting specific heat near the transition as shown in Fig. 3b for the pristine and B Φ =4 T irradiated sample no. 1, respectively. The height of the cusp-like anomaly of sample no. 1 before irradiation (pristine) is ~24 mJ per mol K 2 . After irradiation, the height of the C/T anomaly is slightly suppressed, which can be attributed to a fractional loss of the superconducting material due to the formation of amorphous damage tracks. The transition temperature as revealed by specific heat does not change appreciably with irradiation, in agreement with the magnetic characterization, shown in Fig. 1d,e . 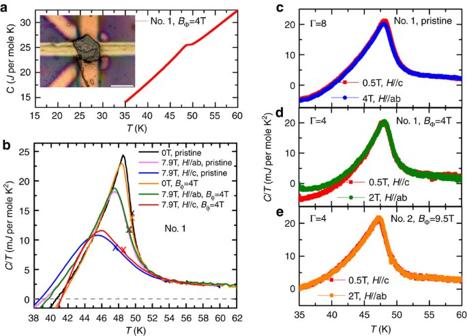Figure 3: Heat capacity and superconducting anisotropy of irradiated SmFeAsO0.8F0.15. (a) Temperature-dependent specific heat of sample no. 1 irradiated to a matching field ofBΦ=4 T. The anomaly due to the superconducting transition near 49 K is clearly seen. The inset shows sample no. 1 with a size ~120 × 90 × 6 μm3placed on top of the ac micro-calorimeter. (b) The electronic heat capacity anomaly nearTcfor pristine sample no. 1 (before irradiation) and after irradiation (BΦ=4 T). The crosses mark the transition temperature as determined from the inflection point of. (c–e) Temperature-dependent specific heat at fixed fields forH||c andH||ab to determine the superconducting anisotropyγ. The ratio of the two orthogonal fields for which theC/Tcurves coincide is the anisotropyγ. Figure 3: Heat capacity and superconducting anisotropy of irradiated SmFeAsO 0.8 F 0.15 . ( a ) Temperature-dependent specific heat of sample no. 1 irradiated to a matching field of B Φ =4 T. The anomaly due to the superconducting transition near 49 K is clearly seen. The inset shows sample no. 1 with a size ~120 × 90 × 6 μm 3 placed on top of the ac micro-calorimeter. ( b ) The electronic heat capacity anomaly near T c for pristine sample no. 1 (before irradiation) and after irradiation ( B Φ =4 T). The crosses mark the transition temperature as determined from the inflection point of . ( c – e ) Temperature-dependent specific heat at fixed fields for H ||c and H ||ab to determine the superconducting anisotropy γ . The ratio of the two orthogonal fields for which the C/T curves coincide is the anisotropy γ . Full size image The superconducting anisotropy can be directly obtained by comparing the resulting heat capacity anomaly at T c when the magnetic field is applied along the c-axis and ab-plane of the crystal. As shown in Fig. 3c , the specific heat data for 0.5 T//c and 4.0 T//ab coincide, revealing a superconducting anisotropy of γ ~8 in the pristine SmFeAsO 0.8 F 0.15 crystal. Similarly, in the irradiated samples with doses of B Φ =4 T and B Φ =9.5 T, the temperature-dependent C/T curves at 0.5 T//c overlap with those at 2.0 T//ab, corresponding to an anisotropy of γ ~4 ( Fig. 3d,e ). This result indicates that the incorporation of a low density of columnar defects reduces the superconducting anisotropy of SmFeAsO 0.85 F 0.15 by one half without changing the transition temperature. This tailoring of the anisotropy reduces the Ginzburg number and thereby enhances the irreversibility line and vortex pinning in irradiated SmFeAsO 0.8 F 0.15 . Our results can be qualitatively accounted for in a model based on anisotropic scattering by columnar defects. In the case of a dilute concentration of scattering centres, point defects mix all momentum states equally, whereas extended defects preserve the momentum along certain directions [29] . For columnar defects, the momentum along the column’s axis is preserved, which is the c-axis in our case. Therefore, after irradiation the electron mean free path l along the c-axis remains the same, whereas l in the ab-plane decreases due to additional scattering from the columns. This can be qualitatively described as and , where and l c represent the c-axis electron mean free path prior and post irradiation. Likewise, and l ab denote the in-plane mean free paths. l irr is the average distance travelled by an electron between two consecutive scattering events from two columns. The anisotropy parameter γ is defined as, where the upper critical fields and are determined in Ginzburg–Landau theory through the in-plane and out-of-plane coherence lengths ξ ab and ξ c (ref. 30 ), and . For the qualitative description given here, we consider identical electron bands or the dominance of one major band in a two-band superconductor, which reduces to the one-band scenario for the upper critical field [31] , [32] . The change in anisotropy induced by the anisotropic scattering due to columnar defects can be expressed in terms of the change of the coherence lengths for both the clean and dirty limits. As presented in more detail in the Supplementary Notes 1 and 2 , the anisotropy parameter γ for a single-band superconductor in the clean limit can be expressed as here γ 0 and denote the anisotropy and mean free path of the unirradiated sample, is the BCS (Bardeen-Cooper-Schrieffer) (or Pippard) coherence length, and is the inverse of the pre-irradiation coherence length. Correspondingly, the anisotropy parameter γ for a single-band superconductor in the dirty limit reads Equations 2 and 3 reveal for both limiting cases that the additional electron scattering by columnar defects, represented by l irr , leads to a reduction of the superconducting anisotropy. As shown in Supplementary Fig. S1 , γ decreases rapidly with increasing defect at low concentrations and levels off at higher concentrations. These results are qualitatively consistent with our experimental observation that at higher defect concentration the anisotropy does not decrease any further within the uncertainties. A quantitative description of the data will require precise knowledge of the relation between l irr and the number of columns and a microscopic modelling of the electron scattering induced by these defects, which are beyond the ambit of this paper. In any case, by incorporating columnar defects along the c-axis, the thermodynamic superconducting anisotropy can be reduced. The rate of reduction with increasing irradiation-induced columnar defects is determined by the number of pre-existing defects, carrier density and the scattering potential of the columnar defects. As the in-plane and out-of-plane upper critical fields are given by and , the reduction of ξ ab brought by anisotropic electron scattering causes a larger enhancement of than of as is directly shown in Fig. 3b for sample no. 1. The enhancement of dH c2 / dT is 2 for fields along the c-axis and 1.2 for fields applied in the plane. The crosses in Fig. 3b mark the superconducting transition temperatures that correspond approximately to the inflection points of C/T according to pervious analysis of the specific heat data of SmFeAsO 1− x F x (ref. 16 ). A reduction of the anisotropy after heavy-ion irradiation with virtually unchanged T c was also observed in 122-compounds. For example, the anisotropy of Ba 0.6 K 0.4 Fe 2 As 2 is reduced from 2.5 to 2.1 after 1.4 GeV Pb-ion irradiation to a dose of B Φ =21 T (ref. 10 ); heavy-ion-irradiated SrFe 2 (As 1− x P x ) 2 shows an anisotropy change from 1.6–1.5 to 1.2–1.3 (ref. 33 ). The comparatively small reduction of anisotropy in the FeAs-122 materials can be attributed to the initial low anisotropy and the discontinuous morphology of the damage tracks [10] . Similar phenomena could be expected in high- T c cuprates, MgB 2 and other anisotropic superconductors. Very limited attention has been paid to the reduction of the superconducting anisotropy due to correlated defects in these materials. In the case of cuprates, any change of H c2 is convoluted with a reduction of T c , whereas the high conductivity of MgB 2 and of most conventional superconductors has prevented the creation of columnar defects with heavy-ion irradiation [34] . For iron-based superconductors, their semimetal property and weak gap anisotropy [2] enable us to tune the anisotropy via heavy-ion irradiation. We expect other poor-metallic and fully gapped type II superconductors to follow our predictions and demonstrate tailored anisotropy as well. This general phenomenon is important for the application of new superconducting materials. The low anisotropy, high critical current and high T c indicate that optimal-doped SmFeAsO 1− x F x may be the best iron-based superconductor for application. Recent progress in SmFeAsO 1− x F x thin film synthesis has provided the premise for fabricating high-quality films using appropriate substrates [13] , [14] . Further improvement of the performance of these films can be expected when columnar-type defects are incorporated. Experiences accumulated over the past decades on creating self-assembled columnar defects in cuprates films [35] via chemical synthesis could help promote similar critical current enhancement in iron-based superconducting films. In this respect, SmFeAsO 1− x F x -based superconducting products with performance comparable to the state-of-the-art of cuprates can be expected. Specific heat measurement We applied a membrane-based steady-state ac micro-calorimeter to measure the calorimetric effect of submicrogram single crystals. It utilizes a thermocouple composed of Au-1.7% Co and Cu films deposited onto a 150-nm-thick Si 3 N 4 membrane as a thermometer. SmFeAsO 0.8 F 0.15 crystals with a size ~100 × 100 × 6 μm 3 were mounted on the thermocouple using Apiezon N grease. An ac-heater current at low frequency (<200 Hz) is adjusted such as to induce oscillations of the sample temperature of 50–200 mK. Critical current measurement The Hall sensor is based on a two-dimensional electron gas GaAs/AlGaAs heterostructure. The Hall-bar array was fabricated by photolithography and chemical etching. The active area is 5 × 5 μm 2 and the sensitivity is 0.27 Ω per Gauss. The low temperature magnetization was measured by a SQUID (Quantum Design) magnetometer with a resolution down to 2 × 10 −8 emu. For both Hall sensor and SQUID measurements, the magnetic field was applied in a step mode and the magnetic responses were measured after a 10-s stabilization time. J c determination using the MO images A high spatial-resolution (down to 1 μm) MO imaging technique was used to map the magnetic induction component, B z , normal to the crystals’ ab-plane. It is based on the Faraday rotation of polarized light in a garnet indicator film placed on top of the sample. The field profile of the trapped flux, B z ( x ) allows us to estimate the critical current density either by numerically integrating Biot–Savart’s law for the supercurrent flow pattern inside the sample or by using an approximate expression for the normal component of the magnetic induction in elongated rectangular thin samples. here, t =6 μm is the thickness of the sample, a is width and z 0 the gap between the MO indicator film and the sample surface. z 0 is obtained from the ratio of the maximum B z at the centre and minimum negative B z near the sample edge , which for a known sample geometry is a unique function of z 0 (ref. 36 ). In our case, k ~10 gives the indicator position z 0 ~10 μm and the critical current density ~10 5 A cm −2 , in good agreement with estimates of J c from the M(H) loops. How to cite this article: Fang, L. et al . Huge critical current density and tailored superconducting anisotropy in SmFeAsO 0.8 F 0.15 by low-density columnar-defect incorporation. Nat. Commun. 4:2655 doi: 10.1038/ncomms3655 (2013).